Engineered probioticEscherichia colican eliminate and preventPseudomonas aeruginosagut infection in animal models Bacteria can be genetically engineered to kill specific pathogens or inhibit their virulence. We previously developed a synthetic genetic system that allows a laboratory strain of Escherichia coli to sense and kill Pseudomonas aeruginosa in vitro . Here, we generate a modified version of the system, including a gene encoding an anti-biofilm enzyme, and use the probiotic strain Escherichia coli Nissle 1917 as host. The engineered probiotic shows in vivo prophylactic and therapeutic activity against P. aeruginosa during gut infection in two animal models ( Caenorhabditis elegans and mice). These findings support the further development of engineered microorganisms with potential prophylactic and therapeutic activities against gut infections. Bacterial infections are a major cause of morbidity and mortality in clinical settings; their impact is exacerbated by the epidemic-like emergence of resistant strains [1] . In addition, antibiotic therapies can eliminate beneficial microbes and lead to the persistence of resistant strains. With growing interest in the importance of the regulatory roles played by microbiota in human health, studies are revealing potential means by which native microbial communities can be exploited to our advantage, thereby providing strategic approaches for managing infections. On the basis of advances in genome engineering and on our understanding of pathogenesis, a microbe-based pathogen-specific antimicrobial strategy that detects and targets infectious pathogens with precision can be envisioned. Probiotics, such as Escherichia coli Nissle 1917, are microorganisms that confer beneficial physiological or therapeutic activities. For example, some probiotics can alleviate intestinal inflammation and irritable bowel syndrome, strengthen host innate immune functions or protect the intestinal barrier against pathogens [2] , [3] , [4] . Further, probiotics can prevent colonization of the human intestinal tract by pathogenic E. coli [5] , [6] . A few studies have exploited engineered probiotics for therapeutic purposes, including site-specific expression and delivery of biomolecules that target bacterial and viral infections [7] , [8] , [9] , [10] , [11] or as adjuvants to pharmacological therapy [12] . However, the majority of such studies have been validated in vitro , and only a few have been evaluated for therapeutic efficiency using in vivo models [13] , [14] , [15] , [16] . Here, we evaluate the efficacy of an engineered probiotic strain against Pseudomonas aeruginosa infection in two in vivo infection models. Although the lungs are a major site of infection by this opportunistic pathogen in immune-deficient patients [17] , [18] , [19] , the intestinal tract is considered to be an important reservoir of P. aeruginosa [20] for opportunistic infections in neutropenic and immunocompromised patients [21] , [22] , [23] , and the presence of this pathogen in the intestinal tract facilitates hematogenous spread to the lungs [24] . In addition to the initiation of respiratory infections from the GI tract, P. aeruginosa gut infection is also responsible for increased mortality in gut-derived sepsis and bacteremia [25] , [26] and causes inflammatory bowel diseases including typhlitis and Shanghai fever [27] . Furthermore, colonization of the GI tract by P. aeruginosa in low-birth-weight infants leads to severe necrotizing enterocolitis and a significant increase in mortality [28] . We previously showed that an engineered microbe can be reprogrammed to detect a specific pathogen ( P. aeruginosa ) by detection of its secreted autoinducer N-acyl homoserine lactone (AHL) and to respond by inducing its own lysis (driven by lysin E7), thus releasing an anti- P. aeruginosa toxin, pyocin S5. The study demonstrated efficient pathogen-specific killing activity in in vitro co-cultures [29] . Here, in addition, we have employed an anti-biofilm enzyme, dispersin B (DspB), to promote the destabilization of mature biofilms to achieve a more apt and physiologically relevant treatment. DspB is naturally produced by Actinobacillus actinomycetemcomitans and hydrolyses 1,6- N -acetyl-D-glucosamine, which is known to stabilize biofilm formation and increase biofilm integrity [30] . Plasmids provide a common framework for synthetic circuits. They are typically retained under the pressure of an antibiotic selection marker, but this presents a potential risk for horizontal gene transfer of the antibiotic resistance to other bacteria. To address this issue, we introduced an auxotrophic marker in E. coli Nissle; the vector-host combination consists of an E. coli Nissle Δ alr Δ dadX strain that requires D-alanine for growth and a plasmid providing the wild-type copy of alr in trans to complement the deletion. The dadX and alr genes encode two alanine racemases that catalyse the interconversion of D-alanine and L-alanine; the D-enantiomer is used in the construction of the peptidoglycan layer of bacterial cell walls. We tested the system in vivo using Caenorhabditis elegans and murine infection models. In both systems, the engineered probiotic E. coli Nissle autonomously executes diagnostic and therapeutic activities that efficiently reduce a pre-colonized P. aeruginosa infection. Furthermore, the engineered probiotic strain exhibited prophylactic activity by conferring specific protection against P. aeruginosa infection. Engineering E. coli Nissle for optimal in vivo expression In E. coli Nissle, the alr and dadX genes encode alanine racemases, which are essential enzymes in D-alanine metabolism [31] , [32] . D-Alanine is an essential building block of Gram-negative peptidoglycan; when both the alr and dadX genes are inactivated, cells become dependent on exogenous D-alanine for survival [31] . We exploited this obligate requirement for alanine racemase to develop an alr -dependent vector-host system in E. coli Nissle ( Fig. 1a ). We introduced gene deletions using a previously described method [33] ; the resulting Nissle Δ alr Δ dadX strain (referred to as EcN hereafter) required D-alanine for growth. For complementation, an alr+ plasmid (pEaaK) was constructed by introducing the native alr gene promoter and Shine–Dalgarno (SD) sequences from wild-type Nissle into the BglBrick backbone [34] ( Supplementary Fig. 1A ). EcN complemented with pEaaK grew in the absence of D-alanine, and its growth rate and viability were comparable to that of wild-type Nissle ( Fig. 1a ). Furthermore, protein expression and plasmid retention in antibiotic-free medium was greatly improved in the pEaaK-containing Nissle (EcN) compared to wild-type Nissle ( Fig. 1a ; Supplementary Fig. 1D ). 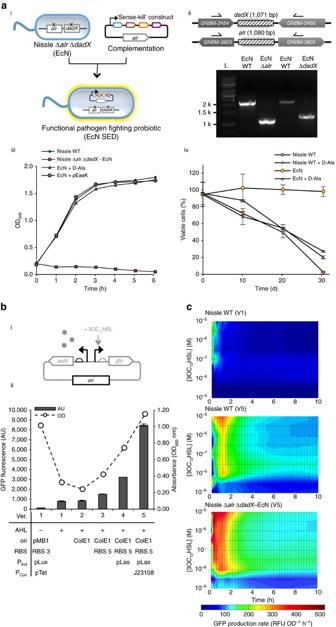Figure 1: Development of optimal cellular host and genetic element systems for a functional probiotic strain. (a) (i) Vector-host system created in theE. coliNissle strain by auxotrophic complementation to stabilize plasmid retention. The ‘Sense-Kill’ construct comprises of: lasR (blue), pyocin S5 (brown), E7 lysis protein (orange) and DspB (purple) (Supplementary Table 1). (ii) The chromosomal deletion ofalranddadXinE. coliNissle was confirmed by PCR. Genes flanking the deleted region are indicated by their annotated gene names:GNBM-2454(D-amino acid dehydrogenase small subunit),GNBM-2456(cell volume regulation protein A),GNBM-3803(ribosyl nicotinamide transporter, PnuC-like),GNBM-3805(hypothetical protein). (iii) Growth of strain EcN (Nissle ΔalrΔdadX) in the presence of exogenousD-alanine (50 μg ml−1) or in the presence of complementary vector (pEaaK;Supplementary Fig. 1). The microtiter plate assay was performed in triplicate wells; the mean and s.e.m. (error bars) from three experiments are shown. (iv) Plasmid retention was tested by culturing wild-type Nissle (non-auxotrophic) and EcN (auxotrophic) cells containing plasmid pEaaK (which includes a kanamycin resistance gene) in the absence of antibiotic and in the presence or absence of exogenousD-alanine in minimal medium. Cell viability in the presence of kanamycin was used to infer plasmid retention and expression. The mean and s.e.m. (error bars) from three experiments are shown. (b) (i) Optimization of the regulatory components of the sensing system (highlighted in black in the circuit diagram) was performed. (ii) The effects of several variations in the regulatory components on GFP expression and bacterial growth were assessed. The mean and s.e.m. (error bars) from three experiments are shown. (c) GFP production per cell over time at different 3OC12-HSL inducer concentrations in Nissle and EcN cells containing the reporter construct. The optimized circuit (V5) showed a lower threshold for 3OC12-HSL detection and sustained expression in the new vector-host system. Figure 1: Development of optimal cellular host and genetic element systems for a functional probiotic strain. ( a ) (i) Vector-host system created in the E. coli Nissle strain by auxotrophic complementation to stabilize plasmid retention. The ‘Sense-Kill’ construct comprises of: lasR (blue), pyocin S5 (brown), E7 lysis protein (orange) and DspB (purple) ( Supplementary Table 1 ). (ii) The chromosomal deletion of alr and dadX in E. coli Nissle was confirmed by PCR. Genes flanking the deleted region are indicated by their annotated gene names: GNBM-2454 (D-amino acid dehydrogenase small subunit), GNBM-2456 (cell volume regulation protein A), GNBM-3803 (ribosyl nicotinamide transporter, PnuC-like), GNBM-3805 (hypothetical protein). (iii) Growth of strain EcN (Nissle Δ alr Δ dadX ) in the presence of exogenous D -alanine (50 μg ml −1 ) or in the presence of complementary vector (pEaaK; Supplementary Fig. 1 ). The microtiter plate assay was performed in triplicate wells; the mean and s.e.m. (error bars) from three experiments are shown. (iv) Plasmid retention was tested by culturing wild-type Nissle (non-auxotrophic) and EcN (auxotrophic) cells containing plasmid pEaaK (which includes a kanamycin resistance gene) in the absence of antibiotic and in the presence or absence of exogenous D -alanine in minimal medium. Cell viability in the presence of kanamycin was used to infer plasmid retention and expression. The mean and s.e.m. (error bars) from three experiments are shown. ( b ) ( i ) Optimization of the regulatory components of the sensing system (highlighted in black in the circuit diagram) was performed. (ii) The effects of several variations in the regulatory components on GFP expression and bacterial growth were assessed. The mean and s.e.m. (error bars) from three experiments are shown. ( c ) GFP production per cell over time at different 3OC 12 -HSL inducer concentrations in Nissle and EcN cells containing the reporter construct. The optimized circuit (V5) showed a lower threshold for 3OC 12 -HSL detection and sustained expression in the new vector-host system. Full size image Due to the ColE1 ori used for pEaaK, the level of alanine racemase expressed might cause an additional metabolic burden [35] , [36] , [37] or potentially affect cell wall synthesis. The expression of alr did not result in a discernible deficit in cell growth, nor did it impede cell-lysis mediated by the E7 protein ( Supplementary Fig. 1B ). Interestingly, it was further noted that the expression of exogenous alanine racemase by our alr + plasmid resulted in a slightly higher growth rate at low pH comparable to that found in a gastric environment ( Supplementary Fig. 1C ). As supplementation of cultures of wild-type Nissle with excess D-alanine also resulted in an improved growth rate, it is postulated that the phenomenon is a result of a higher level of alanine racemase expression compared to the wild-type. We reconfigured this new Nissle strain in our previously described ‘Sense-Kill’ genetic system [29] . It was noted that considerable reduction in GFP expression of the sensing genetic system occurred when the alr + plasmid containing previous GFP reporter system was introduced to wild-type E. coli Nissle ( Fig. 1b,c ). As the recombinant protein expression shows a certain strain-context dependence, genetic components regulating expression in response to the quorum sensing molecule, 3OC 12 HSL, have been systematically optimized for expression in EcN (D-alanine auxotrophic E. coli Nissle) and incorporated into our alr+ vector ( Fig. 1b , Supplementary Fig. 2 ). When the cells were induced with QS molecules and the rates of expression and cell growth were observed over time, the optimized system resulted in a lower threshold of 3OC 12 HSL detection (from 1 μM to 10 nM) and prolonged robust expression of alanine racemase upon induction ( Fig. 1c ). The heat map shows the rate of expression (Fluorescence/OD 600nm /time); the optimized system (V5) was found to produce a more rapid response and a higher rate of GFP expression upon induction than the other systems. The rate of production persisted for ∼ 2 h, followed by an extended period of lower expression. It is possible that the observed reduction in expression after 2 h is caused by the reallocation of cellular resources to favour cellular growth and essential protein expression over orthogonal expression [35] , [36] , [37] . Engineered E. coli Nissle against various stages of P. aeruginosa To evaluate the new strain with improved autoinducer sensitivity coupled with more robust downstream expression, the engineered EcN with anti-microbial and anti-biofilm activity was tested against P. aeruginosa . To add an anti-biofilm activity to the ‘Sense-Kill’ construct, dispersin B (DspB) was expressed and tested for glycosyl hydrolase activity. In Fig. 2a , it can be seen that the glycosyl hydrolase activity of the cells increased linearly with time after induction. The corresponding biofilm dispersal activity is also shown. The revised killing circuit, therefore, consists of previously demonstrated P. aeruginosa -specific bacteriocin, the S5 pyocin and E7 lysis proteins [29] , and the new anti-biofilm enzyme, DspB, in an alanine auxotroph (denoted EcN SED); all of these are actuated in an autonomous manner in response to autoinducers secreted by P. aeruginosa . P. aeruginosa constitutively expressing GFP was co-cultured with EcN SED at various starting cell ratios based on OD 600 values. The growth rate of the cells, as determined based on constitutive GFP expression ( Supplementary Fig. 3A ), shows a significant reduction at equivalent starting OD 600 of EcN SED compared to its lysis control, EcN E7. Further viability assays confirmed the observed reduction in growth rate to be a result of efficient killing of the pathogen in this system. When converted to actual colony-forming units ( Supplementary Fig. 3B ), this ratio demonstrates that a significantly higher degree of inhibition was achieved at a lower ratio of engineered EcN cells to the targeted P. aeruginosa cells; under these conditions, a single-EcN cell was seemingly able to kill three P. aeruginosa cells. To provide appropriate controls for EcN SED, lysis control groups (E7 (EcN E7), S5 and E7 (EcN SE), DspB and E7 (EcN dspB)), non-lytic controls (EcN wild-type (WT) and the EcN Sensor mutant, which contains S5, E7 and DspB with inactivated lasR ), were included in the experiments; the results of the control experiments are summarized in Supplementary Fig. 4 . In preventing biofilm formation and killing P. aeruginosa cells, EcN SE and EcN SED show the greatest reduction in viable cells, resulting in a greatly decreased number of cells available to form microcolonies ( Fig. 2b ). We note, however, that EcN SE expressing S5 was unable to penetrate mature biofilms, precluding a reduction in biofilm mass or in the number of biofilm-encapsulated cells. In addition, although EcN dspB was able to degrade mature biofilms, it did not inhibit biofilm formation or reduce the number of biofilm-encapsulated cells. EcN SED, however, which expresses both S5 and DspB, was able to disassemble mature biofilm structures, resulting in the efficient killing of potentially antibiotic-resistant cells encapsulated within the biofilm matrix (an 80% reduction compared to untreated controls; Fig. 2c,d ). 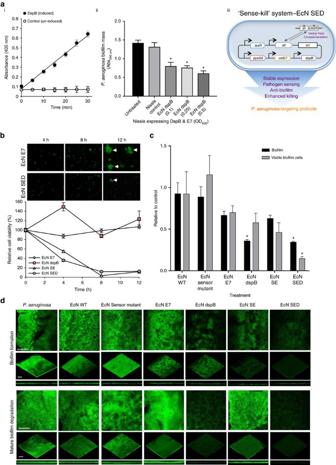Figure 2:In vitrofunctional assays of the engineered probiotic strain. (a) (i) Glycosyl hydrolase activity of DspB with 4-nitrophenyl-N-acetyl-β-D-glucosaminide as substrate. The optical density at 405 nm (OD405 nm) is proportional to the amount of 4-nitrophenolate released in the reaction. (ii) Anti-biofilm activity of DspB expressed by the varying number of EcN cells (OD600 nm) against matureP. aeruginosabiofilm. EcN cells expressing DspB & E7 under quorum sensor are termed ‘EcN dspB’; the change in biofilm biomass was quantified by crystal violet staining. ‘Untreated’ refers to matureP. aeruginosabiofilm. The Nissle control isP. aeruginosabiofilm treated with wild-type EcN cells. The mean and s.e.m. (error bars) from three experiments are shown. * indicates statistical significance (Studentt-test,P<0.05) compared to Untreated and to the Nissle control. (iii) Schematic representation of engineered EcN with the new ‘Sense-kill’ killing circuit, EcN SED (S5 pyocin, E7 lysis protein and Dispersin B), in the auxotrophic vector-host complementation system to produce an optimizedP. aeruginosa-targeting probiotic. (b)P. aeruginosaviability at the indicated time points of co-culture with EcN SED in comparison with lysis control (E7), EcN dspB and EcN expressing S5 & E7 (EcN SE). The data are presented as relative cell survival ofP. aeruginosacells in each treatment group compared to theP. aeruginosacontrol group at each time point. Small aliquots of each co-culture were taken at the indicated time points for microscopic observation. The arrow indicates formation of microcolonies. (c) Anti-biofilm activity was measured by quantifying biofilm mass (by crystal violet staining) and viable biofilm cells (by cell viability counting) after treating mature biofilm with engineered EcN cells for 6 h. The results are shown relative to theP. aeruginosacontrol groups. The mean and s.e.m. (error bars) from three experiments are shown. * indicates statistical significance at an alpha value of <0.05 by one-way ANOVA with the Bonferroni multiple comparisons test. (d)P. aeruginosabiofilm containing the GFP expression vector was grown on 8-well chambered glass slides for 48 h; the biofilm was subsequently treated with the engineered EcN for 6 h and visualized by confocal laser scanning microscopy (CLSM).P. aeruginosawas co-cultured with engineered EcN for 20 h to evaluate its effect on biofilm formation. Images were reconstructed from biofilm Z-stacks (30-μm thickness) using ImageJ. The scale bars represent 100 μm. Figure 2: In vitro functional assays of the engineered probiotic strain. ( a ) (i) Glycosyl hydrolase activity of DspB with 4-nitrophenyl-N-acetyl-β- D -glucosaminide as substrate. The optical density at 405 nm (OD 405 nm ) is proportional to the amount of 4-nitrophenolate released in the reaction. (ii) Anti-biofilm activity of DspB expressed by the varying number of EcN cells (OD 600 nm ) against mature P. aeruginosa biofilm. EcN cells expressing DspB & E7 under quorum sensor are termed ‘EcN dspB’; the change in biofilm biomass was quantified by crystal violet staining. ‘Untreated’ refers to mature P. aeruginosa biofilm. The Nissle control is P. aeruginosa biofilm treated with wild-type EcN cells. The mean and s.e.m. (error bars) from three experiments are shown. * indicates statistical significance (Student t -test, P <0.05) compared to Untreated and to the Nissle control. (iii) Schematic representation of engineered EcN with the new ‘Sense-kill’ killing circuit, EcN SED (S5 pyocin, E7 lysis protein and Dispersin B), in the auxotrophic vector-host complementation system to produce an optimized P. aeruginosa -targeting probiotic. ( b ) P. aeruginosa viability at the indicated time points of co-culture with EcN SED in comparison with lysis control (E7), EcN dspB and EcN expressing S5 & E7 (EcN SE). The data are presented as relative cell survival of P. aeruginosa cells in each treatment group compared to the P. aeruginosa control group at each time point. Small aliquots of each co-culture were taken at the indicated time points for microscopic observation. The arrow indicates formation of microcolonies. ( c ) Anti-biofilm activity was measured by quantifying biofilm mass (by crystal violet staining) and viable biofilm cells (by cell viability counting) after treating mature biofilm with engineered EcN cells for 6 h. The results are shown relative to the P. aeruginosa control groups. The mean and s.e.m. (error bars) from three experiments are shown. * indicates statistical significance at an alpha value of <0.05 by one-way ANOVA with the Bonferroni multiple comparisons test. ( d ) P. aeruginosa biofilm containing the GFP expression vector was grown on 8-well chambered glass slides for 48 h; the biofilm was subsequently treated with the engineered EcN for 6 h and visualized by confocal laser scanning microscopy (CLSM). P. aeruginosa was co-cultured with engineered EcN for 20 h to evaluate its effect on biofilm formation. Images were reconstructed from biofilm Z-stacks (30-μm thickness) using ImageJ. The scale bars represent 100 μm. Full size image Engineered E. coli Nissle in P. aeruginosa -infected C. elegans A simple infection model was established in C. elegans to assess the ability of the engineered EcN to treat P. aeruginosa infection. The nematodes were infected with P. aeruginosa expressing GFP before treatment with engineered EcN SED or with the EcN controls. Gut infections and nematode survival rates were monitored. The infectivity of P. aeruginosa was first established as observed by its accumulation in the digestive tract ( Fig. 3a ). Pathogen-specific activation of ingested EcN SED was further verified by constructing EcN expressing RFP under the control of a genetically encoded sensing system ( Fig. 3b ). Sensor-specific activation was confirmed by the lack of downstream expression when the sensor was inactivated; in this case, EcN with the sensor mutation resulted in survival comparable to that produced by treatment of P. aeruginosa -infected nematodes with wild-type EcN. The ability of the pathogen to kill the nematodes was measured by determining the half-maximal lethal time (the time required to kill 50% of the nematodes, LT 50 ) and the survival rate. In addition, changes in the localization of P. aeruginosa were observed via fluorescence microscopy. 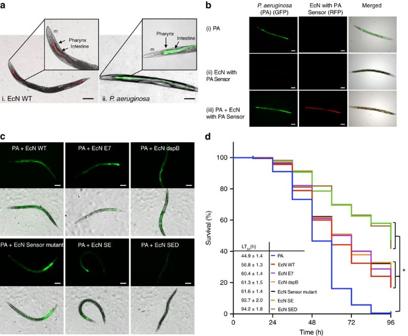Figure 3: Evaluation of the engineered probiotic strain in aC. elegansinfection model. (a) Fluorescence images ofC.elegansshow the localization of (i) wild-type Nissle expressing mRFP1; (ii)P. aeruginosa(PA) expressing GFP. m=mouth. The scale bars represent 100 μm. (b)C. eleganswere given the following for 24 h and viewed by fluorescence microscopy: (i)P. aeruginosa(constitutively expressing GFP) alone; (ii) EcN expressing RFP in the presence of AHL (PA sensor device with RFP); (iii)P.aeruginosafollowed by EcN with PA Sensor (for 4 h) before viewing. The scale bars represent 100 μm. (c) At 24 h post-infection, the nematodes were divided into the following treatment groups; untreated (PA); treated with engineered EcN SED and its control that expresses either E7 alone, S5 & E7 only (SE), DspB & E7 (dspB) or Sensor mutant (disrupted lasR with S5, E7 and dspB gene intact). Representative images of nematodes treated with all the variants of EcN are shown to demonstrate the clearance ofP. aeruginosa(GFP). The scale bars represent 100 μm. (d) The survival rate of each treatment group was quantified until all the nematodes in the infection group had died (96 h). The significance of the results was determined by the Mantel–Haenszel log-rank test followed by Bonferroni’s correction. Statistically significant differences in survival among the groups were not observed. The data from three independent experiments are shown (n=80–100). *P<0.001. Figure 3: Evaluation of the engineered probiotic strain in a C. elegans infection model. ( a ) Fluorescence images of C . elegans show the localization of (i) wild-type Nissle expressing mRFP1; (ii) P. aeruginosa (PA) expressing GFP. m=mouth. The scale bars represent 100 μm. ( b ) C. elegans were given the following for 24 h and viewed by fluorescence microscopy: (i) P. aeruginosa (constitutively expressing GFP) alone; (ii) EcN expressing RFP in the presence of AHL (PA sensor device with RFP); (iii) P . aeruginosa followed by EcN with PA Sensor (for 4 h) before viewing. The scale bars represent 100 μm. ( c ) At 24 h post-infection, the nematodes were divided into the following treatment groups; untreated (PA); treated with engineered EcN SED and its control that expresses either E7 alone, S5 & E7 only (SE), DspB & E7 (dspB) or Sensor mutant (disrupted lasR with S5, E7 and dspB gene intact). Representative images of nematodes treated with all the variants of EcN are shown to demonstrate the clearance of P. aeruginosa (GFP). The scale bars represent 100 μm. ( d ) The survival rate of each treatment group was quantified until all the nematodes in the infection group had died (96 h). The significance of the results was determined by the Mantel–Haenszel log-rank test followed by Bonferroni’s correction. Statistically significant differences in survival among the groups were not observed. The data from three independent experiments are shown ( n =80–100). * P <0.001. Full size image Initially, any potential effect of EcN cells on the survival of C. elegans was evaluated in comparison to the normal food source, E. coli OP50 ( Supplementary Fig. 5B ). It was observed that the survival of nematodes was not affected by feeding EcN cells. Next, C. elegans were infected with P. aeruginosa followed by EcN cells to assess the anti-pathogenic activity of the engineered EcN cells. Interestingly, an increase in survival was observed when infected nematodes were given any EcN cells (including the controls and all of the variants) compared to the infection control group. We note additionally that there was no clear difference in survival among the control variants of EcN. Importantly, the greatest increase in survival rate occurred in the EcN SE and EcN SED treatment groups; in these groups, the survival time increased >2-fold (LT 50 increased from 44.9 h to 92.7–94.2 h), and ∼ 50% of the nematodes in the EcN SE and SED treatment groups remained alive at 96 h post-infection, at which time all the infected nematodes in the infection control group had died. The engineered EcN presumably contributed to the improved survival rate by promoting enhanced clearance of P. aeruginosa from the digestive tract, as the greatest extent and frequency of clearance was observed in the EcN SED group ( Supplementary Fig. 5A ). It is notable that although there were differences in the survival of infected C. elegans treated with EcN with and without S5 pyocin, there was no discernible difference in survival or pathogen clearance between the EcN SE and EcN SED C. elegans treatment groups. As the activity of DspB against biofilms was clearly observed in Fig. 2 , it is possible that either the C. elegans infection model is insufficient for evaluating chronic infection (despite our use of a slow-killing mode of infection [38] ) or biofilm formation within C. elegans does not greatly contribute to death in C. elegans . To further verify the presence or absence of beneficial activity of S5 and DspB co-expression, we examined the relevant protein expression levels. EcN SED is faced with a higher metabolic burden than EcN SE because it expresses an additional protein in the face of limited cellular resources [35] , [36] , [37] . Therefore, EcN SEΔD, which expresses inactive DspB, was constructed; this variant effectively serves as a control with the same metabolic burden as EcN SED. This test permits discrimination of the synergistic activity of DspB and S5 ( Supplementary Fig. 5 ). When the expression of S5 pyocin was lowered to the levels observed in the EcN SED system using EcN SEΔD without active DspB as a metabolic control, significantly lower survival of nematodes compared to EcN SE was observed. Because no discernible activity was observed in the presence of DspB alone (EcN dspB), this suggests that DspB may potentiate the activity of S5, resulting in prolonged nematode survival. The in vivo potentiation of S5 and the anti-biofilm activity of DspB were more closely examined in a murine infection model. Engineered E. coli Nissle in a P. aeruginosa -infected murine model Further evaluation of our engineered EcN was conducted in a P. aeruginosa -infected murine model. In this study, a chronic colonization model was used as this allows discrimination of both the cell killing and the biofilm targeting activities that have been engineered into our EcN synthetic biology constructs that, in turn, are evaluated against the pathological processes associated with P. aeruginosa infection. We first tested the ability of P. aeruginosa to establish chronic colonization in the GI tracts of streptomycin-treated mice over a 13-day period ( Fig. 4a ). After a single administration of 10 10 cfu of live cells, the P. aeruginosa count stabilized to ∼ 10 4 to 10 5 cfu g −1 of faeces and colon tissue after 5 days ( Fig. 4a ). Likewise, the ability of EcN to colonize the gut was verified ( Fig. 5b ). When the mice infected with P. aeruginosa were fed engineered EcN SED, a steady decline in the P. aeruginosa count in the faeces was observed; clearance of the bacterial load reached 77% compared to the initial bacterial load before treatment ( Fig. 4b ). Only a minor decline over time was observed in mice fed EcN E7 or other controls such as EcN dspB and EcN SE. Interestingly, animals fed wild-type EcN showed a transient decline in bacterial load that initially resembled the pattern of EcN SED, but this reversed on day 6 ( Supplementary Fig. 6A ). At the end of the experiment, faecal samples and colon tissues were collected for examination ( Fig. 4b ). A reduction in P. aeruginosa levels was observed in the EcN SE and EcN SED treatment groups compared to the infection control group. A minor reduction in P. aeruginosa levels was observed in other EcN treatment groups (that is, wild-type, E7 lysis control, dspB and Sensor mutant), although statistical significance was not achieved (Kruskal–Wallis test with Dunn correction, P >0.01 for all). Because a minor reduction in bacterial load was observed in the EcN control groups, the activity of EcN SE and EcN SED was compared to that of EcN wild-type (non-lysis control) and E7 (lysis control); only EcN SED achieved a statistically significant reduction in P. aeruginosa colonization (Kruskal–Wallis test with Dunn correction). 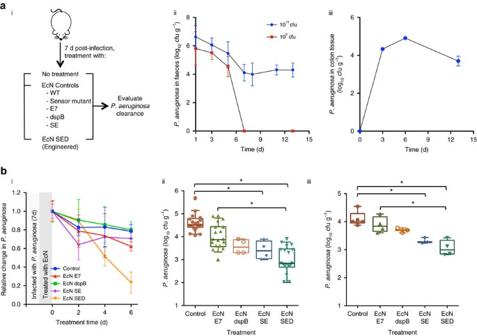Figure 4: Evaluation of the engineered probiotic strain in a mouse infection model. (a) (i) Mice were infected withP. aeruginosa, and gut colonization was studied for 7 days. The mice were then given EcN, andP. aeruginosain faeces was quantified and compared with the infection control group. (ii) Colonization ofP. aeruginosawas assessed by faecal counting of bacteria for two different numbers of cells given by oral gavage. (iii) Colon tissue was homogenized and plated for viability testing to confirm GI infection byP. aeruginosa(1010cfu) over time. (b) (i) The bacterial count relative to averageP. aeruginosainfection at day 0 was tracked over 6 days post-treatment with EcN cells. All EcN expressing E7 are shown for comparison with the lysis controls. Other non-lysis EcN controls (EcN wild-type and Sensor mutant) are shown inSupplementary Fig. 6. (ii–iii) Total viableP. aeruginosacell counts from faecal (ii) and (iii) colon samples at day 6 post-treatment. The data from two independent experiments are shown (n=8–10). *P<0.01 (Kruskal–Wallis test with Dunn correction). Data are presented in box plots with median as centre line, 10 and 90% confidence limits, and minimum and maximum values. Figure 4: Evaluation of the engineered probiotic strain in a mouse infection model. ( a ) (i) Mice were infected with P. aeruginosa , and gut colonization was studied for 7 days. The mice were then given EcN, and P. aeruginosa in faeces was quantified and compared with the infection control group. (ii) Colonization of P. aeruginosa was assessed by faecal counting of bacteria for two different numbers of cells given by oral gavage. (iii) Colon tissue was homogenized and plated for viability testing to confirm GI infection by P. aeruginosa (10 10 cfu) over time. ( b ) (i) The bacterial count relative to average P. aeruginosa infection at day 0 was tracked over 6 days post-treatment with EcN cells. All EcN expressing E7 are shown for comparison with the lysis controls. Other non-lysis EcN controls (EcN wild-type and Sensor mutant) are shown in Supplementary Fig. 6 . (ii–iii) Total viable P. aeruginosa cell counts from faecal (ii) and (iii) colon samples at day 6 post-treatment. The data from two independent experiments are shown ( n =8–10). * P <0.01 (Kruskal–Wallis test with Dunn correction). Data are presented in box plots with median as centre line, 10 and 90% confidence limits, and minimum and maximum values. 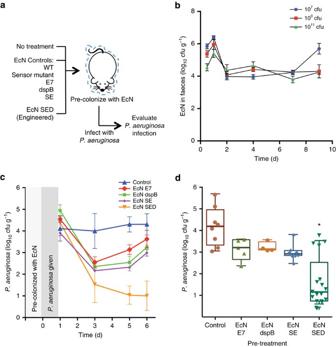Figure 5: Prophylactic activity of engineered EcN againstP. aeruginosainfection. (a) Scheme for pre-colonization of EcN in the GI tract followed byP. aeruginosainfection. (b) Colonization of EcN was assessed by faecal counting of bacteria as a function of time in animals that received different numbers of cells by oral gavage. (c) The level ofP. aeruginosawas tracked over 6 days after giving 1010cfu of the pathogen to each group of pretreated mice. (d) Total viableP. aeruginosacell counts from faecal samples at day 6 post-infection. The data from two independent experiments are shown (n=5–10). *P<0.01 (one-way ANOVA with Bonferroni correction for multiple comparisons). Data are presented in box plots with median as centre line, 10 and 90% confidence limits, and minimum and maximum values. Full size image Figure 5: Prophylactic activity of engineered EcN against P. aeruginosa infection. ( a ) Scheme for pre-colonization of EcN in the GI tract followed by P. aeruginosa infection. ( b ) Colonization of EcN was assessed by faecal counting of bacteria as a function of time in animals that received different numbers of cells by oral gavage. ( c ) The level of P. aeruginosa was tracked over 6 days after giving 10 10 cfu of the pathogen to each group of pretreated mice. ( d ) Total viable P. aeruginosa cell counts from faecal samples at day 6 post-infection. The data from two independent experiments are shown ( n =5–10). * P <0.01 (one-way ANOVA with Bonferroni correction for multiple comparisons). Data are presented in box plots with median as centre line, 10 and 90% confidence limits, and minimum and maximum values. Full size image Next, we evaluated the prophylactic activity of our engineered EcN SED against the onset of infection ( Fig. 5 ). Because our engineered EcN SED is activated only in the presence of P. aeruginosa (via the AHL), it should behave in a manner consistent with wild-type Nissle in the absence of the pathogen. This was a fundamental premise in our initial design concept. The colony counts of EcN and EcN SED in pretreatment samples were consistently similar to each other (not shown). Mice were given EcN SED or the respective EcN controls and subsequently subjected to P. aeruginosa infection. After 6 days of infection, the extent of P. aeruginosa gut colonization was evaluated. Our fully engineered EcN SED provided the greatest protection; in animals treated with EcN SED, lower P. aeruginosa cell counts were observed than in the infection alone group (3.2 log 10 (cfu g −1 )). A low-level of protection (for example, 1–1.5 log 10 reduction) was observed in the other pretreatment groups (wild-type, E7 lysis control, dspB, Sensor mutant and SE), although statistical significance was not achieved (one-way ANOVA with Bonferroni multiple comparisons test, significance achieved when P <0.008). Administration of EcN SED resulted in 98% inhibition of P. aeruginosa infection compared to pretreatment with wild-type EcN. Furthermore, consistent with the results of the C. elegans study, the absence of protection against P. aeruginosa infection by EcN SE or EcN dspB alone supports the synergistic efficacy of combining anti-microbial and anti-biofilm enzymes to target the two bacterial physiological states (that is, planktonic and biofilm) that are present during the initial phase of P. aeruginosa infection. In this work, we demonstrated both prophylactic and therapeutic efficacy of a functional probiotic microbe in vivo against P. aeruginosa infection. The probiotic Nissle strain used in this work has been engineered to achieve highly sensitive and enhanced pathogen-activated expression in non-selective conditions. This arrangement enhanced the stability of the high-copy-number plasmid in the absence of the conventional antibiotic resistance genes that are typically required for plasmid retention, while ensuring sufficient expression of our genetic circuit to produce strong killing capacity. Notably, as the auxotrophic strain containing the Δ alr Δ dadX mutations did not survive in medium devoid of D-alanine without the alr+ plasmid, we suggest that the auxotrophic mutation offers a means of strain biocontainment. When combined with the introduction of the cell-lysis mechanism to the engineered host cells, these features potentially enable a double layer of safety/containment. That is, the engineered cells may promote their own clearance after executing their programmed functionalities in the presence of the pathogen or when the expression construct is lost. The prophylactic and antimicrobial effects of the engineered Nissle strain against P. aeruginosa infection were demonstrated in two animal models. The engineered cells were able to sense the pathogen and accelerate bacterial clearance from the gut in both model systems, and bacterial clearance was visually demonstrated in C. elegans . On the basis of both infection models, although Nissle alone may exhibit beneficial effects against P. aeruginosa , significant clearance occurred only in the presence of the antimicrobial and anti-biofilm proteins (S5 and DspB) in our engineered strain. We also observed that the initial clearance activity that occurred in C. elegans during the first 20 h in the presence of the engineered cells and over a 3- to 4-day period in mice seemed to reflect the eventual survival rate or the extent of clearance of P. aeruginosa at later time points. This can be explained by the eventual clearance of the bacteria by our engineered cells upon detection of P. aeruginosa due to cell-lysis mediated release of the antimicrobial proteins. This might have prolonged clearance of the pathogen in the EcN SED group beyond 3–4 days post-treatment, but this hypothesis warrants further tests. Whereas the highest activity against P. aeruginosa was demonstrated by EcN SED (S5 and DspB), moderately high activity of EcN SE (S5) was observed in both in vivo models. In the C. elegans model, we did not find significant differences in survival between the EcN SE and SED treatment groups, suggesting that the overall survival benefit conferred by S5 in combination with DspB could be achieved through a higher expression level of S5 alone. However, it is the combination of S5 and DspB that exhibited strong clearance and prophylactic activity against P. aeruginosa . This finding supports the idea that combining anti-microbial and anti-biofilm enzymes produces potentiating activity that enhances pathogen killing efficiency. We note, however, that the current design is based on the ability of the bacterium to detect the pathogen-associated quorum-signal molecule, and this naturally presents a limitation in the form of a detection threshold. This potential limitation could be offset, however, by recognizing that the engineered E. coli can also serve as sentinels or reporters of the pathogen [39] , so that repeated dosing might be signalled and enabled. Furthermore, the current design provides a platform through which the genetic features of individual strains can be reprogrammed to provide other biological functionalities or to combat other pathogens of interest. For this reason, our design exclusively targets pathogens that produce AHL as QS molecules and cells that are susceptible to pyocin S5. Although some P. aeruginosa strains are reported to carry immunity genes that confer resistance to this bacteriocin [40] , [41] , the modularity of the genetic circuit used in our design provides a foundation for additional functionalities such as the creation of an S5-immunity inactivation construct or one that causes the bacterium to incorporate complementary antimicrobial peptides. Last, we suggest that the autonomous nature of our design offers an advantage over conventional antibiotic drug therapies, as the administration of antimicrobial probiotics does not require that infection-associated symptoms be present. These bacteria could potentially be freely administered for their normal probiotic-associated benefits as part of a normal probiotic regimen, while also providing potential prophylactic activity against opportunistic pathogens. In support of this idea, our animal data demonstrate that the engineered strain is more efficient in preventing the onset of an infection than in fighting a pre-established one. That is, protection was provided by a single dose of engineered probiotics administered 7 days before exposure to the pathogen. We anticipate that the duration of protection provided by an engineered probiotic would depend on the ability of the cells to remain in the gut, as well as on many other factors. In the mouse intestine, stable colonization by the Nissle strains for periods of up to 3 weeks was observed [5] , [42] ; hence, a single dose of engineered probiotic could potentially provide weeks of protection against the onset of a P. aeruginosa infection. Strains and media All cloning and characterization experiments were performed in E. coli TOP10 (Invitrogen, Carlsbad, CA, USA) unless otherwise stated. Commercial Luria–Bertani (LB) was used as the medium for cloning unless otherwise stated. Kanamycin (30 μg ml −1 ) was added to the culture medium for antibiotic selection where appropriate. P. aeruginosa In7, a clinical isolate that is sensitive to S5 pyocin, was used throughout this study [43] . The probiotic E. coli Nissle 1917 was obtained from Mutaflor (Canada). Generation of deletion mutant and plasmid generation Chromosomal sequences comprising the targeted genes alr and dadX were replaced using the Wanner Lambda Red Gene Disruption kit from the Coli Genetic Stock Center [33] . The primers used for construction of the deletion mutants are listed in Supplementary Table 2 . Mutant candidates were tested for the loss of the target gene by PCR. In addition, mutants were sequenced for genotype confirmation and tested for growth phenotype. The medium was supplemented with D-alanine (50 μg ml −1 ) for the growth of the Δ alr Δ dadX strain (not carrying the alr+ plasmid). The genetic constructs developed in this study were assembled using standard synthetic biology protocols [44] and introduced into the vector pBbE8K (ref. 34 ), which was modified to include a ColE1 replication origin, alr for auxotrophic complementation, and FRT-flanked KanR , (herein referred to as pEaaK). A GFP expression cassette was cloned into pEaaK, and both wild-type and EcN deletion strains were transformed with the plasmid. The transformed cells were grown in tryptone broth in the absence of antibiotic selection and diluted 10,000-fold into fresh medium every 24 h over a 30-day period. GFP expression and KanR phenotype were measured at 10-day intervals as indicators of plasmid retention. Characterization of GFP expression constructs with 3OC 12 -HSL Single colonies of E. coli containing the constructs were inoculated into LB. After overnight growth, the cultures were diluted into fresh LB to a low OD and allowed to incubate further to OD 600 of 0.5. The cultures were then transferred to clear polystyrene 96-well plates in triplicate 200-μl aliquots for induction with homoserine lactone, 3OC 12 -HSL (AHL; Sigma-Aldrich) at varying molar concentrations in 10-fold increments from 10 −9 M to 10 −5 M for 6 h. The plate was incubated at 37 °C with moderate shaking in a microplate reader (Biotek Instruments, USA) and assayed for green fluorescence (excitation; 485 nm and emission; 528 nm). Time-series fluorescence and OD 600 data were obtained over a period of 6 h. The relative GFP production rate was defined as the ratio of background subtracted green fluorescence to OD 600 value. The results obtained from constructs expressed in the Nissle wild-type and the double mutant (Nissle Δ alr Δ dadX —EcN) strains were plotted in MATLAB. Enzyme assay of DspB protein expressed in Nissle A synthetic substrate, 4-nitrophenyl-N-acetyl-β-D-glucosaminide, was used to test the enzymatic activity of DspB. A supernatant was prepared by inducing the expression of DspB and E7 in Nissle for 4 h with 100 nM AHL at an OD 600 of 0.6. Under these conditions, the cells lyse due to E7 expression, releasing DspB into the supernatant. Enzyme reactions were carried out in a 100-μl volume containing 4 mM substrate in PBS buffer and 10 μg ml −1 cellular supernatant; the change in absorption of the supernatant at 405 nm due to the release of p-nitrophenolate was immediately measured. The protein concentration of the supernatant was determined using a standard Bradford assay. Assay for biofilm detachment of P. aeruginosa biofilm treated with engineered EcN Bacterial biofilms were formed by immersing the pegs of a modified polystyrene microtiter lid (catalogue no. 4,45,497; Nunc TSP system) [45] into a 96-well microtiter plate in which each well had been filled with 150 μl of medium containing a single-cell suspension of P. aeruginosa at an OD 600 of 0.05. The plates were incubated at 37 °C for 24 h. The wells were rinsed with PBS, DspB supernatant or engineered EcN (E7 and SED) was added to each well, and the plates were incubated for an additional 4 h. The wells were washed thrice with PBS; the bacteria that remained attached to the surface were stained with crystal violet (0.1% w/v), rewashed under running tap water and dried. The amount of bio-film mass was quantified by destaining the bio-films for 20 min with 95% ethanol and then measuring the absorbance of the crystal violet solution at 595 nm. To assess the number of viable cells within the biofilm, previously published methods were adopted [46] in which the pegs were transferred onto a biofilm recovery plate (a flat-bottom microtiter plate containing antibiotic-free medium). The recovery plate was centrifuged at 805 g for 20 min, and the collected cultures were processed for counting of colony-forming units. Cell viability testing of co-cultured engineered EcN and P. aeruginosa Overnight cultures of P. aeruginosa (bearing a plasmid that conferred constitutive expression of GFP; pMRP9-1) [47] , and engineered Nissle were diluted and harvested at the exponential phase. EcN containing the constructs (E7 or SED) were added to P. aeruginosa cultures (final OD 600 0.2) in appropriate ratios. As P. aeruginosa In7 constitutively expresses GFP from the plasmid, GFP fluorescence was detected using a microplate reader over time to measure the growth retardation. EcN containing the E7 construct (EcN-E7) served as the negative control for EcN SED. For cell viability assays, aliquots of In7 in the mixed culture were quantified by colony-forming unit (cfu) counting on carbenicillin-selective agar plates at regular intervals ranging from 4 to 12 h. Percentage survival of P. aeruginosa was tabulated relative to EcN-E7. Microscopy of biofilms Mixed bacterial cultures of GFP-expressing P. aeruginosa and engineered EcN (SED and its control variants) were cultured in 8-well chamber slides (SPL Lifesciences) in antibiotic-free medium. The biofilm that developed on the glass slides after 18–20 h of growth was rinsed in PBS, dried and visualized using an LSM 510 confocal laser scanning microscope (Zeiss, Jena, Germany). The collected Z-stack biofilm images were reconstructed using ImageJ software. Likewise, biofilm detachment images were prepared after treating the mature biofilms (obtained at 24–48 h of bacterial growth) with engineered EcN for 6 h. The same procedures were repeated with other control variants of EcN as negative controls. Caenorhabditis elegans killing assay The C. elegans strain AU37 used in this study was obtained from the Caenorhabditis Genetic Center ( http://www.cbs.umn.edu/cgc ). AU37 is a pathogen-sensitive strain that exhibits temperature-sensitive sterilization. All nematode-related maintenance protocols were performed according to Powell and Ausubel (ref. 48 ). The worms were allowed to grow at 16 °C for maintenance or at room temperature for sterility or for assays. The pathogenicity killing assay was performed with modifications. Adult nematodes were infected on slow-killing plates (SKPs) containing a P. aeruginosa (with pMRP9-1) bacterial lawn for 24 h. They were then washed off the plates with M9 buffer, collected by centrifugation, and washed two additional times in M9 buffer containing 200 μg ml −1 kanamycin followed by resuspension in M9 buffer. The nematodes were then transferred to SKP plates containing an E. coli bacterial lawn for treatment. The nematodes were observed under fluorescence microscope, and the percentage (%) survival of C. elegans was tabulated. At least three replicates of ∼ 100 worms were carried out. The half-maximal lethal time (LT 50 ) for each treatment was modelled in MATLAB and calculated as described in ref. 38 . For imaging and GFP fluorescence measurement, the nematodes were first anesthetized with 1.5 mM sodium azide (NaN 3 ), then placed on agar and imaged for GFP fluorescence. The fluorescence intensity of 10–20 worms from each treatment group was quantified using ImageJ. Representative individuals were photographed to illustrate the localization of the bacteria. Animal model Studies were performed using 6- to 8-week-old female ICR mice in accordance with international ethical guidelines. All procedures were conducted under IACUC guidelines and in conformity with protocols approved by the SingHealth Institutional Animal Care and Use Committee (2013/SHS/810). Outbred female ICR mice (6–8 weeks old) were given drinking water containing streptomycin sulfate (2 mg ml −1 ) and penicillin (1,500 U penicillin G ml −1 ) for 4 days to eliminate residing facultative bacteria. After 1 day of rest, food was withdrawn overnight, and a single dose of P. aeruginosa (10 10 cfu) in 20% sucrose solution was administered to the mice via oral gavage. Stool samples were collected at the indicated time points and homogenized in 1 ml of 1% protease peptone, serially diluted in this medium and plated on cetrimide agar containing carbenicillin to measure levels of GI colonization. Selection was made against P. aeruginosa harbouring pMRP9.1 plasmid. The mice were randomly subdivided into various EcN treatment groups (wild-type, E7 lysis control and SED-engineered); treatment was given via oral gavage (10 10 cfu). Viability assays of the animals’ faeces were subsequently performed to evaluate the kinetics of clearance of viable P. aeruginosa from the GI tract. Enumeration was performed in a blinded fashion in which the treatment information was unknown. For the prophylactic model, the mice were fed EcN containing pEaaK plasmid or its derivatives (10 10 cfu) in 20% sucrose solution and GI colonization of EcN before P. aeruginosa infection was verified by viability assays of the faeces, using kanamycin for selection. On day 6, the mice were challenged with P. aeruginosa (10 10 cfu), and their subsequent GI colonization was monitored by counting P. aeruginosa in faeces. Each colonization experiment was performed at least twice with 5–10 mice with essentially identical results. Pooled data from at least two independent experiments are presented in the figures. Statistics and reproducibility of results All microtiter plate assays (GFP reporter and biofilm assays) were performed in triplicate wells; the triplicate samples exhibited <10% variation in absorbance and fluorescence values. All assays were performed 2–3 times with similarly significant differences in the quantified values. Results are presented as mean±s.e.m., unless stated otherwise. Student’s t -test and one-way ANOVA were used for statistical analysis involving two groups or multiple experimental group comparisons, respectively. When the sample distributions were not normal, a nonparametric Kruskal–Wallis test was performed. Bonferroni’s correction was performed for multiple comparisons with the significance level α value set to 0.05. The Kaplan–Meier method was applied using GraphPad Prism software to obtain the survival fractions of infected C. elegans treated with variants of EcN. The statistical differences between the survival rates of the EcN-treated groups and the infection control group were determined using the Mantel–Haenszel log-rank test. Data availability The authors declare that all relevant data supporting the findings of this study are available within the article and its Supplementary Information Files or from the corresponding author on request. How to cite this article: Hwang, I. Y. et al . Engineered probiotic Escherichia coli can eliminate and prevent Pseudomonas aeruginosa gut infection in animal models. Nat. Commun. 8, 15028 doi: 10.1038/ncomms15028 (2017). Publisher’s note: Springer Nature remains neutral with regard to jurisdictional claims in published maps and institutional affiliations.